Bio-inspired detoxification using 3D-printed hydrogel nanocomposites Rationally designed nanoparticles that can bind toxins show great promise for detoxification. However, the conventional intravenous administration of nanoparticles for detoxification often leads to nanoparticle accumulation in the liver, posing a risk of secondary poisoning especially in liver-failure patients. Here we present a liver-inspired three-dimensional (3D) detoxification device. This device is created by 3D printing of designer hydrogels with functional polydiacetylene nanoparticles installed in the hydrogel matrix. The nanoparticles can attract, capture and sense toxins, while the 3D matrix with a modified liver lobule microstructure allows toxins to be trapped efficiently. Our results show that the toxin solution completely loses its virulence after treatment using this biomimetic detoxification device. This work provides a proof-of-concept of detoxification by a 3D-printed biomimetic nanocomposite construct in hydrogel, and could lead to the development of alternative detoxification platforms. Owing to their inherent small size and flexibility in rational design and preparation, functional nanoparticles have shown potential applications in effective detoxification [1] , [2] , [3] , [4] , [5] , [6] . Pore-forming toxins (PFTs) that can damage cellular membrane are key virulence factors of pathologies resulting from animal bites/stings and bacterial infections [7] , [8] , [9] . Conventional detoxification platforms such as antisera [10] , monoclonal antibodies [11] and small-molecule inhibitors [12] are hard to completely neutralize toxins because of their limited capability of blocking the whole PFTs’ molecule. Meanwhile, over 80 PFTs have been identified, displaying diverse molecular structures and distinctive epitopic targets [13] . The commonly used antidotes target the specific molecular structures of PFTs; thus, customized treatments are required for different toxins. Recent advancements in the field have spurred the development of nanoparticles that can efficiently bind PFTs and neutralize their toxicity in vivo [1] , [2] , [4] . Although poisoned patients may benefit from these strategies, intravenous administration of nanoparticles causes nanoparticle-toxin accumulation in the liver [1] , thus leading to the risk of secondary poisoning especially in liver-failure patients [14] . Despite these challenges, cleaning blood by adsorption of toxins to retrievable nanoparticles provides an alternative strategy for detoxification. Meanwhile, similar to injection of antidotes, it is clinically approved to remove toxins by in vitro devices [15] . In this work, we demonstrate that polydiacetylene (PDA) nanoparticles can attract, capture and sense PFTs. Taking advantages of three-dimensional (3D) biomimetic structure in enrichment, separation and detection [16] , [17] , [18] , we develop a bio-inspired 3D detoxification device by installing PDA nanoparticles in a precise 3D matrix with modified liver lobule configuration via an advanced 3D printing technology, that is, dynamic optical projection stereolithography (DOPsL). The DOPsL technology utilizes a digital mirror array device (DMD) to generate dynamic photomasks that can be translated into a 3D complex structure through layer-by-layer photopolymerization of biomaterials. The DOPsL technology has great efficacy and versatility in fabricating 3D complex geometries for functional devices and even artificial tissues [19] , [20] , [21] , [22] . As schematically presented in Fig. 1 , this bio-inspired 3D device is designed to efficiently collect and sense PFTs for future detoxification applications. 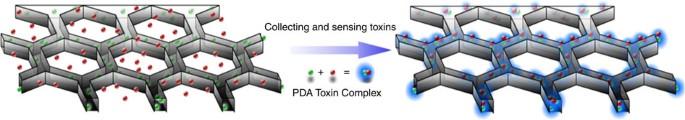Figure 1: Bio-inspired 3D detoxification device. PDA nanoparticles (green) are installed in PEGDA hydrogel matrix (grey) with liver-mimetic 3D structure fabricated by 3D printing. The nanoparticles attract, capture and sense toxins (red), while the 3D matrix with modified liver lobule structure allows toxins to be trapped efficiently. This biomimetic 3D detoxifier has promising clinical application for detoxification by collecting and removing toxins. Figure 1: Bio-inspired 3D detoxification device. PDA nanoparticles (green) are installed in PEGDA hydrogel matrix (grey) with liver-mimetic 3D structure fabricated by 3D printing. The nanoparticles attract, capture and sense toxins (red), while the 3D matrix with modified liver lobule structure allows toxins to be trapped efficiently. This biomimetic 3D detoxifier has promising clinical application for detoxification by collecting and removing toxins. Full size image Neutralizing toxin using PDA nanoparticles To develop functional nanoparticles for constructing a 3D detoxification device, we used PDA nanoparticles derived from self-assembly of 10, 12-pentacosadiynoic acid (PCDA; Supplementary Fig. 1 ). Specifically, blue and colourless PDA nanoparticles with vesicle structure were prepared by ultraviolet irradiation of self-assembled colourless PCDA nanovesicles [23] , [24] . The nanoparticle surface is made of a π-conjugated polymer with alternating double- and triple-bond groups in the main polymer chain. The cell membrane-mimicking surface functions to attract, capture and neutralize toxins owing to the interactions between PDA and toxins. Binding toxins to PDA nanoparticles disrupts the extensively delocalized enyne backbones of molecularly ordered PDA side chains, thus inducing a fluorescence enhancement (none-to-fluorescence) as well as colour change (blue-to-red), as schematically illustrated in Fig. 2a . 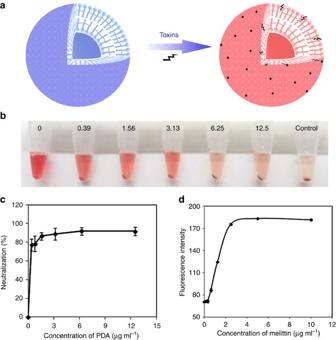Figure 2: Neutralization of toxins by PDA nanoparticles. (a) Schematic presentation of the interaction between PDA nanoparticles and toxins. PDA nanoparticles with cellular membrane-mimetic surface can attract and capture toxins, accompanied with fluorescence change (none-to-fluorescent). (b) Centrifuged RBCs after incubation with normal saline (control) or melittin (5 μg ml−1) mixed with different concentrations of PDA nanoparticles. (c) Quantified efficiency of neutralizing the haemolytic activity of melittin (5 μg ml−1) by PDA nanoparticles. (d) Intensity of red fluorescence of PDA nanoparticles (20 μg ml−1) that were exposed to melittin with different concentrations at 37 °C for 30 min. Figure 2: Neutralization of toxins by PDA nanoparticles. ( a ) Schematic presentation of the interaction between PDA nanoparticles and toxins. PDA nanoparticles with cellular membrane-mimetic surface can attract and capture toxins, accompanied with fluorescence change (none-to-fluorescent). ( b ) Centrifuged RBCs after incubation with normal saline (control) or melittin (5 μg ml −1 ) mixed with different concentrations of PDA nanoparticles. ( c ) Quantified efficiency of neutralizing the haemolytic activity of melittin (5 μg ml −1 ) by PDA nanoparticles. ( d ) Intensity of red fluorescence of PDA nanoparticles (20 μg ml −1 ) that were exposed to melittin with different concentrations at 37 °C for 30 min. Full size image We evaluated the ability of PDA nanoparticles to capture and neutralize toxins by a red blood cells’ (RBCs) lysis test. A widely studied PFT, melittin, was chosen and mixed with PDA nanoparticles and then added to murine RBCs. The centrifuged RBCs’ solution was incubated with normal saline (as a control) or melittin mixed with PDA nanoparticles at different concentrations, as shown in Fig. 2b . Qualitatively, melittin mixed with more PDA nanoparticles produced a clearer supernatant, indicating that less RBCs were damaged. The neutralization efficiency was quantified via colorimetric readings and is presented in Fig. 2c . The results show that PDA nanoparticles can capture and neutralize melittin in vitro . The melittin-binding capacity of PDA nanoparticles is higher than 1 mmol g −1 . This capacity is greater than that of previously reported protein-adsorbing films [25] , nanofibres [26] and nanoparticles [1] . The neutralization efficiency of PDA nanoparticles is ∼ 92%. We also studied the ability of PDA nanoparticles to sense toxins. As shown in Fig. 2d , the interaction between melittin and PDA significantly enhanced the red fluorescence of PDA nanoparticles. The red fluorescence intensity of PDA increased with the concentration of melittin. Meanwhile, the binding of melittin can also induce a slight colour change of PDA nanoparticles (see Supplementary Fig. 2 ). By using the fluorescence data, we calculated the binding constant between melittin and PDA nanoparticles as 630 M −1 from Langmuir isotherm. Compared with recently reported nanoparticles with 100% neutralization of melittin [1] , [4] , the PDA nanoparticle has a lower binding constant, which may be one of the reasons why PDA nanoparticles cannot achieve 100% neutralization of melittin. To better understand the interaction between PDA nanoparticles and melittin, we performed computer simulations at the molecular level. The optimized structure of PDA is present in Supplementary Fig. 3 . After docking PDA to melittin, nine conformations of complex composed of melittin and PDA were obtained. For all of these conformations, the binding affinities between the two components of the complex are negative, suggesting that PDA possesses the capability to bind melittin. The conformation on the top of the list ( Fig. 3a, I ) has the most negative binding affinity: −1.8 kcal mol −1 . In this conformation, PDA interacts with melittin via its hydrophobic tails (seven, in total) and one polar head ( Fig. 3a, II ). On the other hand, half of 26 residues in melittin interact with PDA. Among these residues, only Thr10, Lys21 and Arg24 are polar residues ( Fig. 3a, III ). An electrostatic interaction between the carboxyl group of one polar head in PDA and the guanidine part of Arg24 in melittin was also observed ( Fig. 3a, I ). The interactions between PDA and melittin were further studied by performing simulated annealing using molecular dynamics (MD). MD simulation can facilitate modelled system to surmount small energy barriers on the potential surface and locate sites of lower potential energy, while dynamic annealing can obtain a minimum energy. As exhibited in Fig. 3b , PDA and melittin adjusted their orientations and approached each other in the simulation, suggesting that PDA can attract melittin in close proximity, followed by capture. Also, we found that interaction with melittin can affect the conformation of PDA, which may explain our experimental findings of fluorescence enhancement and colour change of PDA after incubation with melittin. The last conformation of the modelled system was experiencing simulated annealing and subsequent equilibrium. Moreover, by simulated annealing using MD, the PDA–melittin interaction mode was obtained and presented in Fig. 3c . On the basis of these simulations, we conclude that hydrophobic and electrostatic interactions exist between PDA and melittin, and the former interaction contributes much more than the latter; this in theory supports PDA nanoparticles to capture PFTs. 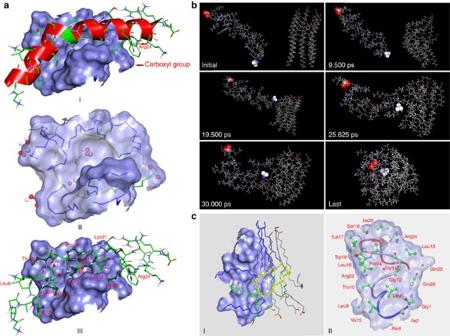Figure 3: Computer simulations on the interactions between PDA and melittin. (a) Simulation results obtained by docking PDA to melittin. I: Conformation of the complex composed of PDA and melittin. The interface is represented with a light blue solid surface and carbon atoms of melittin are coloured with green. Groups that take part in electrostatic interaction have been marked. II: PDA under the interface. Polar heads and hydrophobic tails that interact with melittin are represented with stick. Their carbon atoms are coloured with green and blue, respectively. III: Melittin above the interface. Atoms that interact with PDA are represented with scaled ball and stick and carbon atoms are coloured with dark green. (b) Interactions between PDA and melittin studied by performing simulated annealing using MD. PDA and melittin adjust their orientations and approach each other, followed by forming a complex. The carboxy terminal and amino terminal of melittin are highlighted. (c) PDA–melittin interaction mode obtained by performing simulated annealing using MD. I: PDA on the interaction interface. Polar heads and hydrophobic tails that interact with melittin are represented with stick and coloured with blue and green, respectively. II: Interaction mode of melittin to PDA. Residues that interact with PDA are represented with scaled ball and stick and their carbon atoms are coloured with green. Figure 3: Computer simulations on the interactions between PDA and melittin. ( a ) Simulation results obtained by docking PDA to melittin. I: Conformation of the complex composed of PDA and melittin. The interface is represented with a light blue solid surface and carbon atoms of melittin are coloured with green. Groups that take part in electrostatic interaction have been marked. II: PDA under the interface. Polar heads and hydrophobic tails that interact with melittin are represented with stick. Their carbon atoms are coloured with green and blue, respectively. III: Melittin above the interface. Atoms that interact with PDA are represented with scaled ball and stick and carbon atoms are coloured with dark green. ( b ) Interactions between PDA and melittin studied by performing simulated annealing using MD. PDA and melittin adjust their orientations and approach each other, followed by forming a complex. The carboxy terminal and amino terminal of melittin are highlighted. ( c ) PDA–melittin interaction mode obtained by performing simulated annealing using MD. I: PDA on the interaction interface. Polar heads and hydrophobic tails that interact with melittin are represented with stick and coloured with blue and green, respectively. II: Interaction mode of melittin to PDA. Residues that interact with PDA are represented with scaled ball and stick and their carbon atoms are coloured with green. Full size image Capturing toxin in the 3D-printed hydrogel nanocomposites After confirming the PDA nanoparticles’ ability to attract and capture melittin in solution, we designed a 3D device consisting of a biomaterial hydrogel scaffold to make the nanoparticles retrievable. We used a photocrosslinked poly(ethylene glycol) diacrylate (PEGDA) hydrogel as a 3D matrix. PEGDA is often used in biomedical applications because it is non-toxic, non-immunogenic, favourable to nutrient and oxygen transport, and tunable in its mechanical properties. To chemically link PDA nanoparticles into the networks of PEGDA hydrogel, we synthesized a diacetylene derivative called PCDA-acrylamide (PCDA-A 5 , Supplementary Fig. 4 ). It is based on the diacetylene moiety of PCDA with an extended ethylene oxide spacer arm and an acrylamide functional head group. By mixing PCDA and PCDA-A 5 , the resulting nanoparticles possess acrylamide group on its surface ( Supplementary Fig. 5a ), and can be chemically tethered to the PEGDA hydrogel through addition polymerization ( Fig. 4a ). The nanoparticles have a mean particle size of ∼ 100 nm according to the scanning electron microscope image ( Supplementary Fig. 5b ). The particles’ distribution was determined by dynamic light scattering, as shown in Supplementary Fig. 6a . The nanoparticles have a mean particle size of 110 nm with polydispersity index of 0.23. Meanwhile, the nanoparticles have a zeta potential of −25 mV ( Supplementary Fig. 6b ). Owing to the extremely slow degradation rate of PEGDA network, once chemically immobilized in PEGDA hydrogel, it is difficult for PDA nanoparticles to release into the solution. As shown in Supplementary Fig. 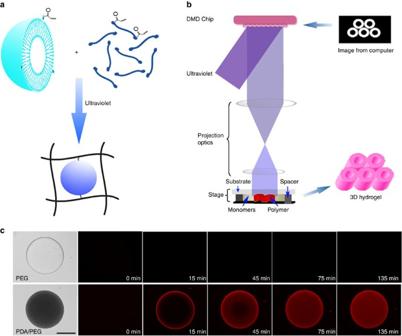Figure 4: Immobilization of PDA nanoparticles in 3D-structured PEGDA hydrogel. (a) Schematic presentation of installing PDA nanoparticles in the network of PEGDA hydrogel. PDA nanoparticles can be chemically linked to the network of PEGDA hydrogel by photocrosslinking PEGDA monomer and acrylamide-modified PDA nanoparticles via addition polymerization. (b) Schematic drawing of the DOPsL method to fabricate 3D-structured PEGDA hydrogel. By rationally designing the masks, PEGDA hydrogel with precise 3D structure can be created. (c) The fluorescence of PEGDA hydrogel of cylindrical shape with or without PDA nanoparticles after incubation with a melittin solution (50 μg ml−1). The fluorescence indicates that melittin is captured by PDA nanoparticles. Scale bar, 50 μm. 7 , no significant amount of PDA nanoparticles were released from the PEGDA hydrogel in 24 h. Figure 4: Immobilization of PDA nanoparticles in 3D-structured PEGDA hydrogel. ( a ) Schematic presentation of installing PDA nanoparticles in the network of PEGDA hydrogel. PDA nanoparticles can be chemically linked to the network of PEGDA hydrogel by photocrosslinking PEGDA monomer and acrylamide-modified PDA nanoparticles via addition polymerization. ( b ) Schematic drawing of the DOPsL method to fabricate 3D-structured PEGDA hydrogel. By rationally designing the masks, PEGDA hydrogel with precise 3D structure can be created. ( c ) The fluorescence of PEGDA hydrogel of cylindrical shape with or without PDA nanoparticles after incubation with a melittin solution (50 μg ml −1 ). The fluorescence indicates that melittin is captured by PDA nanoparticles. Scale bar, 50 μm. Full size image Taking advantages of the photocrosslinkable hydrogel, DOPsL technology, which employs a digital mask and ultraviolet light source for layer-by-layer photopolymerization, was utilized to fabricate 3D PEGDA hydrogels with precise microstructures, as shown in Fig. 4b . As a proof of concept, PEGDA hydrogels with and without PDA nanoparticles were fabricated into simple 3D cylinders and subsequently incubated with melittin solution (50 μg ml −1 ). As shown in Fig. 4c , initially the control PEGDA hydrogel (without nanoparticles) was transparent and non-fluorescent. No colour or fluorescent changes were detected after incubation with melittin. In comparison, PDA nanoparticles incorporated hydrogel appeared opaque (the colour is blue because of the PDA) without fluorescence initially. After incubation with melittin solution (50 μg ml −1 ), however, the composite hydrogel cylinder emanated red fluorescence, which gradually diffused from the surface to the inner part in a time-dependent manner, indicating successful binding of melittin to PDA. Next, we studied the effect of the hydrogel’s specific surface area on the efficiency of capturing toxins. We designed and fabricated three types of 3D posts with the same flower-like projection and length but different diameters, where the thinner post displayed higher specific surface area. As shown in Fig. 5 , melittin can gradually diffuse into all types of post. In the same period, red fluorescence can only be detected on the outer area of the thicker posts while in the thinner posts, the fluorescent signals were also observed in the inner region. On the basis of the previous data that the fluorescent signals correspond to PDA–melittin interaction, the fluorescent signal trends we observed here could imply a modulation of PDA–melittin interactions owing to the specific surface area. The 3D structure containing PDA nanoparticles with a higher specific surface area may be more efficient in enriching toxins. In addition, we found that macromolecules with a higher molecular weight diffuse slower into the PEGDA hydrogel (as shown in Supplementary Fig. 8 ), implying that physical properties such as the porosity of the hydrogel can affect the diffusion of molecules into PEGDA hydrogel, and the PEGDA hydrogel may allow melittin to diffuse faster into the inner structure compared with others macromolecular proteins in the plasma. 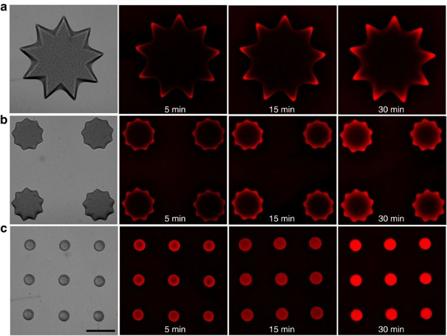Figure 5: Capturing toxin in the 3D-printed hydrogel nanocomposites with different surface patterns. Three types of 3D structural posts with the same flower-like shape and length but different diameters are incubated with melittin solution (50 μg ml−1) for different time at 37 °C. (a) The post with a large diameter. (b) The post with a medium diameter. (c) The post with a small diameter. The red fluorescence implies the PDA and melittin interactions, indicating the site that toxins reach at. Scale bar, 200 μm. Figure 5: Capturing toxin in the 3D-printed hydrogel nanocomposites with different surface patterns. Three types of 3D structural posts with the same flower-like shape and length but different diameters are incubated with melittin solution (50 μg ml −1 ) for different time at 37 °C. ( a ) The post with a large diameter. ( b ) The post with a medium diameter. ( c ) The post with a small diameter. The red fluorescence implies the PDA and melittin interactions, indicating the site that toxins reach at. Scale bar, 200 μm. Full size image Designing the bio-inspired detoxification device To move this surface area-dependent detoxification material to a physiologically relevant design, we integrated the structure of the liver, given its utility in the body’s detoxification. The liver has a hexagonal lobule structure centred around the terminal hepatic vein, which helps to efficiently remove wastes and xenobiotics from the system. We therefore designed a liver-mimetic structure with modified liver lobule topology that allows the toxin to reach the centre of the matrix quickly, as shown in Fig. 6a . Our modified structure has a higher specific surface area than the typical liver lobule structure, which is beneficial for toxins to enter the 3D device effectively. Two types of mask patterns ( Fig. 6b ) were designed and alternatively printed by the DOPsL method layer-by-layer, and finally a liver-mimetic 3D detoxifier was fabricated. After incubated with melittin (50 μg ml −1 ), the 3D microstructure of this detoxifier was observed under a confocal microscope. From the red fluorescence of toxin-bound PDA nanoparticles, the structure of this detoxifier was reconstructed and the results are presented in Fig. 6c . A scanning electron microscope image revealed the multilayer microstructure with modified liver lobule topology ( Fig. 6d ). Meanwhile, we can observe the surface of the matrix with some arrested nanoparticles ( Supplementary Fig. 9 ). Finally, we tested the capability of this detoxifier to capture toxins. Compared with the slab, the liver-mimetic structure makes the detoxifier to neutralize toxins faster, owing to the faster diffusion of toxins into the inner structure ( Fig. 6e ). In Fig. 6f , the RBC solution incubated with melittin treated by our biomimetic detoxifier has a clear supernatant similar to that of the saline control. The red colour of the supernatant in PDA nanoparticle-treated group is more significant than that in the biomimetic detoxifier-treated group. Our 3D biomimetic detoxifier achieved 100% neutralization of toxins while the equivalent amount of free PDA nanoparticles neutralizes 91% toxins, and the PEGDA hydrogel matrix alone has little capacity in neutralizing toxins (shown in Fig. 6g ). Therefore, this biomimetic detoxifier can effectively neutralize toxins, serving as a new technology platform for detoxification. 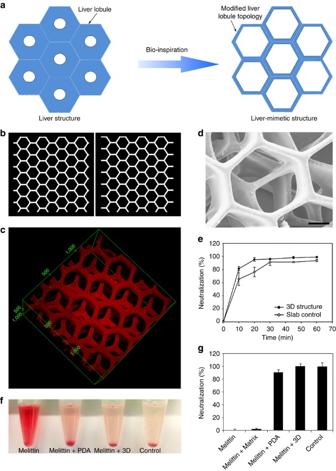Figure 6: The bio-inspired 3D detoxifier. (a) Rational design of the liver-mimetic 3D structure. The modified liver lobule topology allows toxins to enter the 3D matrix efficiently. (b) The masks that are used for printing liver-mimetic 3D structure. By alternatively using these masks in DOPsL technology, a bio-inspired detoxifier with four layers of liver-mimetic structure is created. (c) The 3D structure of the detoxifier measured by laser confocal microscopy. Incubated with melittin (50 μg ml−1, 300 μl), the red fluorescence of PDA allows the reconstruction of the microstructure of the detoxifier in 3D. (d) Scanning electron microscope image of this detoxifier. Scale bar, 50 μm. (e) Dynamic test on the neutralization efficiency with comparison between the liver-mimetic structure (3D structure) and slab control (that is, with the same total volume). After the incubation of melittin solution with detoxifier for different times, the neutralization efficiency was tested by the haemolytic assay. (f) Centrifuged RBCs after incubation with normal saline (control), melittin (5 μg ml−1), detoxifier-treated melittin or PDA nanoparticles-treated melittin. The red colour indicates the cytolysis of RBCs. (g) Neutralization efficiency of the 3D detoxifier. Equivalent amount of PDA nanoparticles is used for comparison. Figure 6: The bio-inspired 3D detoxifier. ( a ) Rational design of the liver-mimetic 3D structure. The modified liver lobule topology allows toxins to enter the 3D matrix efficiently. ( b ) The masks that are used for printing liver-mimetic 3D structure. By alternatively using these masks in DOPsL technology, a bio-inspired detoxifier with four layers of liver-mimetic structure is created. ( c ) The 3D structure of the detoxifier measured by laser confocal microscopy. Incubated with melittin (50 μg ml −1 , 300 μl), the red fluorescence of PDA allows the reconstruction of the microstructure of the detoxifier in 3D. ( d ) Scanning electron microscope image of this detoxifier. Scale bar, 50 μm. ( e ) Dynamic test on the neutralization efficiency with comparison between the liver-mimetic structure (3D structure) and slab control (that is, with the same total volume). After the incubation of melittin solution with detoxifier for different times, the neutralization efficiency was tested by the haemolytic assay. ( f ) Centrifuged RBCs after incubation with normal saline (control), melittin (5 μg ml −1 ), detoxifier-treated melittin or PDA nanoparticles-treated melittin. The red colour indicates the cytolysis of RBCs. ( g ) Neutralization efficiency of the 3D detoxifier. Equivalent amount of PDA nanoparticles is used for comparison. Full size image PDA is a π-conjugated polymer that has been extensively studied as a sensor matrix, because of its colour (blue-to-red) and fluorescence (none-to-fluorescent) changes in response to environmental cues [27] , [28] , [29] , [30] , [31] , [32] . Currently, while synthesis and utilization of DA monomers with new functional groups remains interesting [33] , expanding their utility as functional building blocks to construct 3D supermolecular assemblies enables new and improved applications of PDAs [34] , [35] . 3D PDAs show superior properties such as higher stability, increased surface area and multipoint interaction sites. In this work, a new application of PDA nanoparticles for detoxification was demonstrated. We used computer simulations to understand the molecular mechanism of interaction between PDA and melittin. Moreover, we synthesized PCDA-A 5 functional nanoparticles with alkenyl groups on its surface, followed by chemical immobilization in a photocrosslinked 3D hydrogel using 3D printing. To our knowledge, this is the first attempt to precisely incorporate PDAs in 3D hydrogels with a biomimetic architecture. We specifically used PEG-derived hydrogels for the 3D detoxification device. PEG is well known as a biocompatible and ‘stealth’ material [36] , [37] , and PEG hydrogels have been widely used in biomedical applications such as tissue engineering [38] , drug delivery [39] and in vitro 3D cell culture [40] , [41] . In addition, the pore sizes of the patterned PEG hydrogel can be easily tuned to enable efficient solute exchange [42] and PEG itself is resistant to bio-fouling and non-specific absorption of biomacromolecules in vitro and in vivo [43] . Therefore, PEG hydrogel is an ideal biocompatible matrix for carrying functional nanoparticles, allowing the nanoparticles to function in a controlled 3D space [44] . In this work, PDA nanoparticles are chemically immobilized in a 3D PEG hydrogel and used for collecting and sensing toxins. This idea of incorporating particles into hydrogel for detoxification purposes has been demonstrated by early studies [45] , [46] , [47] . We propose to shape the PEG matrix encapsulated with PDA nanoparticles into a designer structure using 3D printing, a disruptive technology that is finding promising applications in creating unique 3D devices and tissue constructs [48] , [49] . Inspired by the liver structure that contributes to fast substances’ exchange between blood stream and hepatic cells [50] , we fabricated PEG hydrogels into a liver-mimetic structure with modified liver lobule configuration, producing a higher specific surface area than the original liver lobule. This bio-inspired designer 3D structure allows toxins to enter the PEG matrix effectively and interact with these nanoparticles with toxins’ affinity, providing new insight for rationally designing a 3D detoxifier for potential clinical applications in detoxification ex vivo . PFTs are one of the most common peptide toxins. Recently, based on the functional similarity among different PFTs in perforating cellular membranes, an action mechanism-targeted detoxification concept was illustrated [2] , suggesting that cellular membrane-mimetic matrix can be used to capture and neutralize a variety of PFTs. In our work, PDA nanoparticles with a cellular membrane-mimetic surface are developed to attract, capture and sense toxins, followed by immobilization within a liver-mimetic 3D PEG hydrogel matrix, creating a 3D biomimetic detoxifier. Our data show that the toxin’s solution completely lost its virulence in damaging cellular membrane after treatment with the 3D detoxifier. Recently, Hoshino et al. [1] , [4] prepared a library of tailored multifunctional copolymer nanoparticles and demonstrated that their nanoparticles with high binding affinity can achieve 100% neutralization of toxins in vitro , providing a novel method for designing advanced plastic antidotes. Similar to other cellular membrane-mimetic nanoparticles [2] , the PDA nanoparticles can work as artificial cells to efficiently neutralize PFTs, although they cannot achieve 100% neutralization efficiency, possibly because of a low binding constant. Our 3D detoxifier can separate the toxin/PDA complex from cells so that the RBCs are limited to interact with the melittin on the surface of PDA nanoparticles, resulting in an enhanced detoxification efficiency compared with free PDA nanoparticles. In addition, conventional detoxification in intravenous application of nanoparticles shows risk of causing secondary poisoning especially in liver-failure patients, owing to their accumulation in the liver [1] , [2] . Here inspired by the liver microstructure, we demonstrate a liver-mimetic 3D detoxification device that can collect and remove toxins, providing a novel strategy for designing nanoparticle-enabled detoxification treatments. Moreover, the cell-free nature of our detoxifier allows integration of a variety of functionalities and nanoelements in rationally designed microarchitectures. This could lead to many breakthroughs in the development of future detoxification platforms. Materials PEGDA (Mw=700 Da), melittin and PCDA were purchased from Sigma (USA). PCDA was further purified by dissolving in dichloromethane and then filtered to remove polymerized monomers before use. Photoinitiator lithium phenyl-2,4,6-trimethylbenzoylphosphinate was synthesized according to the previous work [22] . Computational simulation The interactions between melittin and PDA were studied using two kinds of computational simulation methods. One is to dock PDA to melittin with the help of AutoDock Vina and the other is to perform simulated annealing using MD ( Supplementary Methods ). Synthesis and identification of PCDA-A 5 The synthesis scheme of PCDA-A v has been presented in Supplementary Fig. 4a . In a 50-ml flask with a stir bar, compound 1 (PCDA, 374 mg, 1.0 mmol) was dissolved in dry CH 2 Cl 2 (10 ml) followed by addition of triethylamine (101 mg, 1.0 mmol) and N , N ′-disuccinimidyl carbonate (256 mg, 1.0 mmol). The reaction solution was stirred at room temperature for 1 h to activate compound 1 , creating active ester 2 . Then, acid 3 (74 mg, 1.0 mmol) was dissolved in dry CH 2 Cl 2 (10 ml), followed by adding triethylamine (101 mg, 1.0 mmol) and N , N ′-disuccinimidyl carbonate (256 mg, 1.0 mmol). The resulting solution was stirred at room temperature for 1 h, and then amine 4 was added. The reaction solution was monitored by liquid chromatography–mass spectrometry. Four hours later, ester 2 was added. The reaction was stirred at room temperature for 4 h, product 5 (PCDA-A 5 ) was found by liquid chromatography–mass spectrometry analysis. The reaction solution was evaporated and the residue was purified by flash column chromatography to produce 84 mg compound 5 as white solid. The yield was 15%. The PCDA-A 5 was identified by 1 H NMR ( Supplementary Fig. 10 ), 13 C NMR ( Supplementary Fig. 11 ) and high resolution mass spectrometer ( Supplementary Fig. 12 ). Preparation of PDA nanoparticles To prepare the PDA nanoparticles, 40 mg of PCDA was added into 8 ml of distilled water, followed by probe sonication for 5 min at ∼ 75 °C. Then, the solution was stored overnight at 4 °C. At last, the solution was irradiated with ultraviolet for 5 min in ice bath, creating blue and non-fluorescence PDA nanoparticles [23] . PCDA-A 5 and PCDA mixed nanoparticles were prepared by sonication of the mixed PCDA-A 5 and PCDA (mass ratio 1:19) in hot water (at about 75 °C). 3D printing via DOPsL The DOPsL set-up illustrated in Fig. 4b was used to fabricate the 3D structures using photopolymerizable polymers [21] . The sliced images of the 3D model were loaded to the DMD chip that can continuously generate optical patterns and expose the photopolymerizable material in a layer-by-layer manner. PEGDA (20 wt%) in H 2 O with 1% lithium phenyl-2,4,6-trimethylbenzoylphosphinate was mixed with PDA particles suspension (5 mg ml −1 ) in an equal volume ratio. The mixture was then loaded to the sample stage of DOPsL and polymerized via patterned ultraviolet exposure to fabricate corresponding 3D structures. The DMD chip used in the set-up is DLP-07 XGA from DLP Technology of Texas Instruments. After the PDA nanoparticles were immobilized, the 3D structure was incubated in PBS for 2 h at 37 °C, and then irradiated by ultraviolet for 5 min to allow the polymerization of PDAs. Efficiency of detoxification Neutralization of the haemolytic activity of melittin by PDA nanoparticles was assayed by a modified standard haemolytic assay procedure [1] , [2] . Melittin (final concentration in RBC suspension was 5 μg ml −1 ) was pre-incubated with the same volume of PDA nanoparticles for 30 min at 37 °C in PBS. The melittin/NP mixture (100 μl) was then added to the RBC solution (2% v/v, 100 μl), followed by incubation at 37 °C for 30 min. Samples were then centrifuged at 800 g for 5 min. The release of haemoglobin was measured by bicinchoninic acid kit. Controls for 0 and 100% neutralization of haemolytic activity consisted of RBCs incubated with 5 μg ml- melittin ( A 0% ) and a RBC suspension with normal saline ( A 100% ), respectively. The percentage of neutralization was calculated according to equation (1): To study the neutralization efficacy of our 3D PDA nanoparticle-enabled detoxifier, 50 μl of melittin (50 μg ml −1 ) was pre-incubated in the device for 60 min at 37 °C. Then, the melittin solution was carefully collected by directly pipetting the melittin solution and washing the device with 200 μl PBS. The resulting 250 μl solution was then added to a 250-μl RBC solution (4% v/v), followed by incubation at 37 °C for 30 min. Finally, the percentage of neutralization was calculated. In addition, the neutralization efficiency of the 3D detoxifier was compared with that of the equivalent amount of PDA nanoparticles or PEGDA hydrogel. Moreover, the dynamic test was performed on the neutralization efficiency with comparison between the liver-mimetic structure (3D structure) and slab control (that is, with the same total volume). After the incubation of melittin solution with detoxifier for different times, the neutralization efficiency was tested by the haemolytic assay. How to cite this article: Gou, M. et al. Bio-inspired detoxification using 3D-printed hydrogel nanocomposites. Nat. Commun. 5:3774 doi: 10.1038/ncomms4774 (2014).